Direct mechanochemical cleavage of functional groups from graphene Mechanical stress can drive chemical reactions and is unique in that the reaction product can depend on both the magnitude and the direction of the applied force. Indeed, this directionality can drive chemical reactions impossible through conventional means. However, unlike heat- or pressure-driven reactions, mechanical stress is rarely applied isometrically, obscuring how mechanical inputs relate to the force applied to the bond. Here we report an atomic force microscope technique that can measure mechanically induced bond scission on graphene in real time with sensitivity to atomic-scale interactions. Quantitative measurements of the stress-driven reaction dynamics show that the reaction rate depends both on the bond being broken and on the tip material. Oxygen cleaves from graphene more readily than fluorine, which in turn cleaves more readily than hydrogen. The technique may be extended to study the mechanochemistry of any arbitrary combination of tip material, chemical group and substrate. Applying heat, pressure or light are common approaches to accelerate a chemical reaction. A less common but highly efficient alternative drives the reaction through direct mechanical stress, often yielding reaction products that are otherwise difficult to synthesize [1] , [2] . Much about mechanochemical reactions remains poorly understood. Macroscale mechanochemical processes such as ball milling and ultrasonic cavitation are often used to drive such reactions [3] , [4] ; however, in situ characterization is difficult and the delivery of precise stresses is not possible. Pulling on individual molecules with atomic force microscope (AFM) [5] tips can rupture bonds with pN resolution, but the technique is limited to molecules long enough to detect rupture and systems where the bonds between tip and sample are stronger than the bond under investigation [6] , [7] , [8] , [9] . There is a need for an experimental system capable of measuring mechanochemical bond scission that can be applied universally to a wide variety of material systems and that produces quantitative information about the chemical reaction occurring. While mechanically induced chemistry is a well-established phenomenon, it has historically been difficult to generate well-defined experiments. For instance, mechanochemical studies with relatively precise control over stresses exist for hard lubricating films such as diamond-like carbon using pin-on-disk tribometers where a millimetre diameter ball continuously rubs against a film [10] . Decades of careful research have shown that the performance of such carbon films depends on multiple factors including the relative amount of sp 2 versus sp 3 carbon centres, surface roughness, the presence of other chemical functional groups, the substrate and the environment. However, despite extensive study, these wear studies have produced only empirical relationships between mechanical load and film chemistry, due in part to poor chemical definition of the starting material, film inhomogeneity and environmental contaminants [10] . Consequently, there has been a growing interest in using nanometre scale, single asperity sliding contacts to probe mechanochemical bond scission at the tip–substrate interface, and recent work has shown volumetric resolution approaching a few atoms [11] , [12] . It remains unclear, however, what role surface topography plays, which bond or bonds are being broken and which properties—length, energy, polarization and so on—of the bond are important. Although the experimental apparatus has been highly developed, what has been lacking is a more defined material system that enables unambiguous identification of the bonds broken, removes the complication of corrugation and allows bonds to be broken singly. While this is difficult to achieve in three-dimensional (3D) crystalline materials, the 2D carbon lattice found in graphene is ideal for mechanochemistry since it is atomically flat, can be produced with exceptional crystalline quality, can be functionalized with a wide range of chemical groups and is easily characterized by conventional surface science techniques [13] , [14] . Chemically modifying graphene markedly alters its optical [15] , electronic [16] and lubricating [17] , [18] properties. It should be noted that while prior work has shown that scanning probes can remove functional groups by locally applying heat [16] , [19] or electronic potential [20] ; mechanochemical cleavage by a scanning probe has not been addressed. Here we introduce an AFM technique to study mechanochemical bond cleavage of arbitrary organic bonds within zeptolitre volumes on chemically modified graphene (CMG) sheets. Monitoring the friction between the tip and graphene provides an in situ method to measure the kinetics of functional group removal and the relative bond strength of the functional groups. The chemical flexibility of graphene enabled us to mechanically cleave several different functional groups including hydrogenated graphene (HG), plasma oxygenated graphene (OG) and fluorinated graphene (FG), and so directly determine how the character of the bond impacts its scission. Moreover, the approach clearly demonstrates that the chemistry of the tip material itself can alter the reaction by altering the required stress for the reaction. Indeed, this robust experimental arrangement enables all the mechanochemical reactants—the tip (Si, Si 3 N 4 and diamond), the functional groups on the film (O, F and H) and the substrate (SiO 2 and Cu)—to be interchanged to measure the reaction kinetics in detail. This technique could be extended to study mechanochemical bond scission of any arbitrary organic bond using any tip–molecule–substrate system. Relating chemical composition to lateral force Mechanochemical cleavage occurred for all systems examined and under a wide range of conditions. 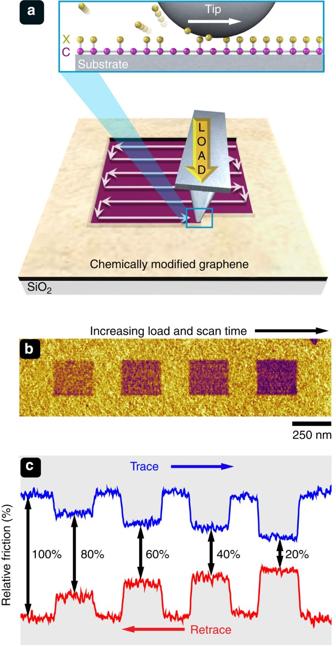Figure 1: Measuring and controlling chemical bond scission on graphene (a) Schematic of the AFM mechanochemical process where a scanning AFM tip with a known normal load removes chemical groups from a graphene sheet and measures the removal with lateral friction measurements. (b) A lateral friction scan on plasma OG with four areas reduced with increasing local contact stress and scan time. The desired friction level was set before mechanochemical processing. (c) A linescan of the four squares showing up to a 5 × reduction in friction due to the removal of oxygen groups. Load and scan time were tuned during the removal process to quickly reach the desired friction reduction, where higher loads and longer scan times led to faster and more complete removal of functional groups. Figure 1a illustrates the process for removing oxygen-rich functional groups from an isolated square region on an OG sheet. Applying loads between 10 and 500 nN with an AFM tip controllably cleaved functional groups from OG, and hundreds of lithographic features ranging in width from 18 nm to over 10 μm were patterned at speeds up to 500 μm s −1 . For the starting OG material, X-ray photoelectron spectroscopy (XPS) showed that most of the functional groups were carbonyls (C=O, 48%) followed by other oxygen bonds (C–OH or C–O– or C–O–C, 30%; O–C=O, 22%; see Methods section for details) [21] . Since the areas for mechanochemical cleavage were carefully chosen away from tears and edges, the bonds cleaved were predominately epoxide and hydroxide groups that reside on the basal plane and not the carbonyl and carboxyl groups, which reside at the graphene edges [22] . Because graphene has lower friction than all the CMGs used, monitoring the friction provided a direct, in situ measure of the local chemistry, as discussed below. Longer scans and higher loads resulted in greater removal of the functional groups, providing a tool to tailor the local surface chemistry exactly. This was achieved by intermittently measuring the friction force during mechanochemical bond cleavage and stopping the reaction at the desired friction, and hence surface concentration, by decreasing the load. For example, Fig. 1b shows a friction force image of four patches where the desired levels of friction were programmed to be 20, 40, 60 and 80% of the original friction value, as indicated by the friction force linescan shown in Fig. 1c . Such cleavage was not observed in previous work on CMG friction measurements likely due to low tip loading, short scan times and surface contamination; although, there is insufficient information present to make contact stress comparisons [23] . Figure 1: Measuring and controlling chemical bond scission on graphene ( a ) Schematic of the AFM mechanochemical process where a scanning AFM tip with a known normal load removes chemical groups from a graphene sheet and measures the removal with lateral friction measurements. ( b ) A lateral friction scan on plasma OG with four areas reduced with increasing local contact stress and scan time. The desired friction level was set before mechanochemical processing. ( c ) A linescan of the four squares showing up to a 5 × reduction in friction due to the removal of oxygen groups. Load and scan time were tuned during the removal process to quickly reach the desired friction reduction, where higher loads and longer scan times led to faster and more complete removal of functional groups. Full size image The measured change in friction directly relates to the mass removed from the surface in the form of covalently bound chemical groups. Previous studies of friction on CMG have established that the added chemical groups interact more strongly with the tip than does the graphene, thus raising the friction [18] , [23] , [24] . Consequently, the relative friction difference between functionalized and pristine graphene is a direct measure of the degree of chemical functionalization, where lower-friction force values correspond to fewer chemical groups attached to the basal plane. This point may be reinforced by noting that the change in friction force is linearly proportional to the volume of functional groups cleaved from the surface and that the ultimate height decrease of 3.7±1.3 Å corresponds roughly to the length of an –OH group ( Supplementary Fig. 1 and Supplementary Discussion , section ‘Friction versus removed mass’). Thus, friction force provides a robust in situ means to track the areal concentration of functional groups bound to the graphene surface. Two additional experiments confirm bond cleavage: Raman spectroscopy shows functional group removal after mechanical processing, and conductivity measurements taken during the removal show increased electronic conductivity as the insulating CMG is converted to more conductive graphene ( Supplementary Fig. 2 and Supplementary Discussion , section ‘Film characterization’). Finally, the basal plane remains intact throughout the experiment, since rupturing the basal plane leads to easily detectible film failure ( Supplementary Fig. 3 ). Bond scission dynamics The removal rate of oxygen-rich groups from OG shown in Fig. 2a was determined by repeatedly scanning a single square and monitoring the monotonic decrease in friction force as a function of cumulative tip dwell time and tip normal load. Tip dwell time depends critically on the contact radius between the tip and surface, so contact radius was routinely measured ( Supplementary Fig. 4 and Supplementary Discussion Calculating tip dwell time and contact stress). For each point in a single reaction curve at one load ( Fig. 2b ), a 250 × 250 nm 2 square region ( N =65,536) was scanned ( Supplementary Movie 1 ). Critically, increasing the applied load significantly increases the mechanochemical reaction rate. 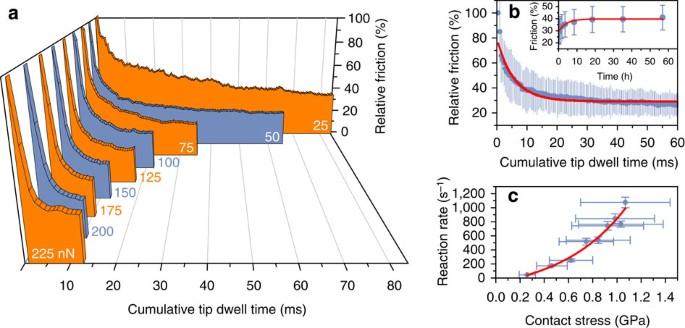Figure 2:In situmeasurement of bond scission dynamics (a) Relative friction force measurements as a function of cumulative tip dwell time for normal loads 25–225 nN, showing an increasing exponential decay rate with increasing normal load. (b) Reaction curve for 50 nN normal load showing the kinetics of bond scission follows an exponential decay typical of a first-order chemical reaction. At low loads, a contamination layer contributes an additional decay term. This contamination layer slowly resorbs over many hours (inset). The error bars are the s.d. of the friction force values for each AFM scan. (c) Reaction rate as a function of measured contact stress, showing an exponential dependence consistent with an atomic-by-atom stress-assisted reaction mechanism. Thexaxis error bars were calculated by propagating uncertainty values from the linear fit of tip contact radius measurements to the calculation of contact stress. Theyaxis error comes from the calculated uncertainty of the exponential fit to the data ina. For a given load, the relative decrease in friction force with tip dwell time was well fit ( R 2 =0.95) with an exponential: Figure 2: In situ measurement of bond scission dynamics ( a ) Relative friction force measurements as a function of cumulative tip dwell time for normal loads 25–225 nN, showing an increasing exponential decay rate with increasing normal load. ( b ) Reaction curve for 50 nN normal load showing the kinetics of bond scission follows an exponential decay typical of a first-order chemical reaction. At low loads, a contamination layer contributes an additional decay term. This contamination layer slowly resorbs over many hours (inset). The error bars are the s.d. of the friction force values for each AFM scan. ( c ) Reaction rate as a function of measured contact stress, showing an exponential dependence consistent with an atomic-by-atom stress-assisted reaction mechanism. The x axis error bars were calculated by propagating uncertainty values from the linear fit of tip contact radius measurements to the calculation of contact stress. The y axis error comes from the calculated uncertainty of the exponential fit to the data in a . Full size image representing a first-order process governed by reaction rate λ 1 . Friction force measurements spanning days after removal of oxygen groups showed a small increase in friction with an exponential rise time of ≈4 h ( Fig. 2b inset), suggesting that the initial rapid decay not captured by the exponential fit may be attributed to adsorbed environmental contaminants that slowly resorb onto the surface after removal, as seen before in carbon systems by Erdemir and colleagues [25] . Additional measurements of friction change behaviour for graphene oxygenated as grown on a copper foil further showed that the change in friction is not due to contaminants from the graphene transfer process ( Supplementary Fig. 5 ). Despite the reversible friction contribution from contaminants, the friction force reduction represented by this term persists indefinitely as a result of permanent removal of functional groups. Fitting equation (1) to the data in Fig. 2a yielded values for λ 1 as a function of applied contact stress ( Fig. 2c ), showing an exponential relationship ( Supplementary Figs 6 and 7 , and Supplementary Discussion , section ‘Calculating tip dwell time and contact stress). Recent work has shown that atomic-scale stress-assisted mechanochemical processes can be modelled with a modified version of the Arrhenius thermal activation model where Δ U act is the energy activation barrier, σ is the applied stress, Δ V act is the activation volume acted on by the stress, k B is Boltzmann’s constant, T is absolute temperature and λ 0 is an effective attempt frequency pre-factor (where reasonable attempt frequencies are based on atomic vibrations in the range 10 13 –10 15 s −1 ; refs 11 , 26 ). Fitting the reaction rate data as a function of applied stress from Fig. 2c at a known temperature (30 °C) resulted in an activation volume of 10.6±1.6 Å 3 and an activation energy of 0.73±0.06 eV. Since we are likely removing hydroxyls and epoxides from the graphene basal plane, the calculated activation volume and activation energy should correspond to removal of these structures. The activation volume is generally held to be the volume over which the stress must dissipate for the reaction to occur. The measured activation volume 10.6±1.6 Å 3 compares favourably with literature values for the volumes of epoxides (13.1 Å 3 ) and for hydroxyls (14.8 Å 3 ), confirming that bonds should be removed one by one as expected [27] . Second, the activation energy of 0.73±0.06 eV is comparable to previous density functional theory calculations, which found a binding energy of 0.67–0.70 eV for hydroxyls on graphene and 1.9–2.7 eV for epoxides on graphene [28] , [29] . Note that because we did not vary the temperature, the value of the activation energy depends on the assumed attempt frequency. Thus, the values for both the activation volume and activation energy are reasonable for the current system, suggesting removal of hydroxyl groups and epoxides from the graphene lattice. Relative bond strength If the bond rupture is purely mechanical, then higher bond strengths should require larger forces to break. We studied the relationship between bond strength and mechanochemical removal by monitoring the friction force on different CMGs while linearly ramping the normal load on the tip between each scan. This is similar to the conventional method for taking friction-load plots. 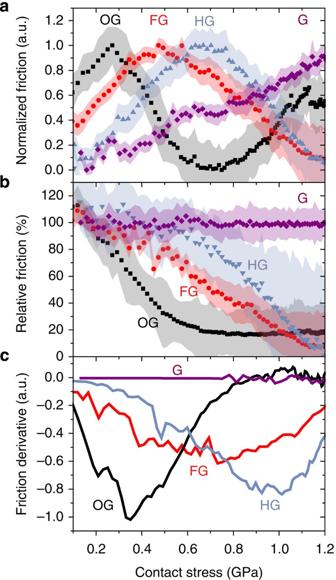Figure 3: Chemical composition changes during a contact stress ramp (a) Normalized friction force as a function of applied contact stress for plasma OG, FG, HG and an unmodified graphene sheet. The error bars were determined from the s.d. of each lateral force scan. (b) Relative friction compared with the CMG sheet outside of the scan area, showing the degree of functional group removal. The data were captured by a tip scanning at a set low load (10 nN) after a scan at the load indicated on the abscissa. The error bars were calculated as the s.d. of lateral force divided by the average lateral force for each data point. (c) Derivative of friction force, where the minima indicate the maximum reduction rate in friction. The data was smoothed using the Savitzky–Golay smoothing algorithm to clearly show the trends. Figure 3a shows the normalized friction force as a function of tip load for pristine graphene such as OG, FG and HG. Pristine graphene gave the expected response, with friction increasing monotonically and approximately linearly with normal load. In contrast, the friction on all the CMG sheets showed an unexpected nonlinear behaviour—at low contact stresses the friction forces increased linearly but then decreased as the functional groups were removed to reveal lower-friction graphene. Once the groups were fully removed, the friction force again increased linearly with normal load. Although this is another example of a ‘negative friction coefficient’, the mechanism here differs significantly from that recently reported by Cannara and colleagues, wherein the wetting of the AFM tip by OG causes sheet delamination and thus higher dissipation at lower loads [17] . Rather, we observed a persistent, repeatable chemical change in the CMG ( Supplementary Fig. 8 and Supplementary Discussion , section ‘Repeatability’). Figure 3: Chemical composition changes during a contact stress ramp ( a ) Normalized friction force as a function of applied contact stress for plasma OG, FG, HG and an unmodified graphene sheet. The error bars were determined from the s.d. of each lateral force scan. ( b ) Relative friction compared with the CMG sheet outside of the scan area, showing the degree of functional group removal. The data were captured by a tip scanning at a set low load (10 nN) after a scan at the load indicated on the abscissa. The error bars were calculated as the s.d. of lateral force divided by the average lateral force for each data point. ( c ) Derivative of friction force, where the minima indicate the maximum reduction rate in friction. The data was smoothed using the Savitzky–Golay smoothing algorithm to clearly show the trends. Full size image Monitoring the relative mass loss from the graphene film as a function of applied stress provides a measure of the strength of the ruptured bonds. After each scan at linearly increasing loads, the friction values for the square and the adjacent nonreduced film were measured at low loads (≈10 nN). Figure 3b uses the ratio of these values to remove any potential effect of tip shape or intermittent contamination. The derivative of this curve ( Fig. 3c ) gives the rate of loss with contact stress and enables the determination of the contact stress required to remove different functional groups. These contact stresses were as follows: 0.37±0.18 GPa for OG, 0.72±0.39 GPa for FG and 0.89±0.21 GPa for HG. The position of these values may be understood by recognizing that the force required to rupture a bond, including thermal energy, must exceed the slope (d E /d x ) of the potential energy curve under extension. Higher bond energies clearly should require greater forces; and it has been suggested that longer bond lengths should require lower forces [3] . Density functional theory calculations of bond energy and bond length exist for each system studied here [28] , [30] and are summarized in Table 1 . The force required to remove each bond can be estimated from the ratios of the bond energy E bond to the bond length l bond given in Table 1 , and the trend in the forces calculated from the density functional theory data corresponds to the observed trend in contact stresses measured here for CMG. The table also demonstrates the importance of bond length since both –H and >O epoxy have comparable energies, but the much shorter bond length of –H increases the required pressure for removal. Clearly, direct measurements of these bond lengths and energies would improve our understanding of these processes, as would refined models to relate the macroscopic quantity of contact stress to atomic interactions between the tip and 2D films. Table 1 Density functional theory calculated bond lengths and binding energies. Full size table Effect of tip material A final benefit of this experimental approach is that the tip can be treated as a reactant in the mechanochemical reaction. Typically, the scanning probe is contaminated by a transfer film; however, as explained above, the presence of transfer films can be quickly detected in this experimental configuration. Consequently, we explored how the chemical nature of the tip, in addition to the stress applied, impacts the reaction. 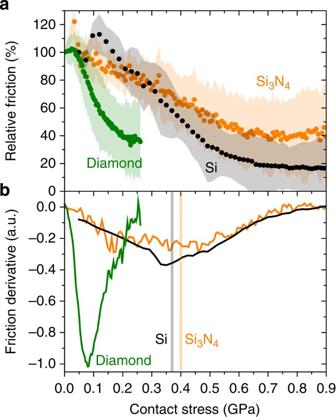Figure 4: The effect of tip material on the local chemical reaction (a) Relative friction drop on OG as a function of contact stress for a diamond (green), silicon (black) and silicon nitride (orange) tip. For reference, the data for Si is the same as forFig. 3. The error bars were calculated as the s.d. of lateral force divided by the average lateral force for each data point. (b) Derivative of the friction decrease for all three tips, showing that the kinetics of oxygen group removal is the same for SiN and Si tips, while the diamond tip removes the oxygen groups with ~4 × lower contact stress. The data was smoothed using the Savitzky–Golay smoothing algorithm to clearly show the trends. Figure 4a shows relative friction reduction as a function of contact stress for silicon, silicon nitride and diamond (Advanced Diamond Technologies, Inc.) tips. As above, Fig. 4b shows the derivative of the friction, revealing the contact stresses for the fastest removal of oxygen groups. Notably, both the Si and Si 3 N 4 tips remove functional groups with the same dependence on contact stress—0.37±0.18 GPa for Si and 0.40±0.23 GPa for Si 3 N 4 . In contrast, the diamond tip drives the reaction at a much lower stress of 0.08±0.02 GPa ( Supplementary Fig. 8 ). This lower reaction barrier suggests that the removal of functional groups from the graphene depends on the tip chemistry, either through direct reaction of the graphene oxygen groups with tip material or through a catalytic process mediated by the surface chemistry of the tip. In the latter case, the silicon, silicon nitride and diamond tips all present hydroxyl groups at their surfaces. However, the acidity of tertiary carbon hydroxyls is quite different from that of silanol hydroxyls, and the possibility exists for acid- or base-mediated hydroxyl removal from the graphene sheet. Alternatively, high stress may promote wear of the diamond tip and activate the hydroxyls on the graphene and tip surfaces, facilitating a redox disproportionation reaction suggestive of the well-known Boudouard reaction [31] . In contrast to previous AFM pulling force measurements on long molecule chains, where the AFM tip is distant from the ruptured bond, here we show that the tip material actively contributes to bond scission. This behaviour helps confirm that a mechanochemical reaction between the tip material and the exposed covalent bond on the graphene is occurring, and provides a route to understanding and quantifying these reactions by simultaneously monitoring wear of both the surface and the tip. Figure 4: The effect of tip material on the local chemical reaction ( a ) Relative friction drop on OG as a function of contact stress for a diamond (green), silicon (black) and silicon nitride (orange) tip. For reference, the data for Si is the same as for Fig. 3 . The error bars were calculated as the s.d. of lateral force divided by the average lateral force for each data point. ( b ) Derivative of the friction decrease for all three tips, showing that the kinetics of oxygen group removal is the same for SiN and Si tips, while the diamond tip removes the oxygen groups with ~4 × lower contact stress. The data was smoothed using the Savitzky–Golay smoothing algorithm to clearly show the trends. Full size image In conclusion, mechanochemical AFM on CMG sheets provides a flexible and powerful new tool to study stress-driven chemistry. Quantitative determinations of the activation energy and activation volumes are directly obtained. The known orientations of the chemical bond relative to the tip and substrate simplify interpretation of the results and would expedite efforts to model the system via density functional theory. More importantly, the tip, the functionalization and the substrate can all be varied, enabling a refined approach in studying arbitrary C–X bonds. Judicious choice of tip material, substrate, chemical functional groups and scanning parameters will provide insight into the reaction pathway occurring under the tip. That is, whether the reaction proceeds under compressive or tensile stress, the effect of substrate [32] and if the tip material acts as a reaction catalyst. Finally, although the work presented here focuses on graphene, this methodology can be applied to any covalently functionalized 2D material, many of which are currently actively studied [33] , [34] , [35] . Material preparation Graphene was grown using chemical vapour deposition on Cu foil substrates [36] in an ‘enclosure’ geometry [37] . The growth was carried out at 1,030 °C for ~1 h with flowing methane ( P CH4 ≈30–50 mTorr) and hydrogen ( P H2 ≈5 mTorr) and subsequently quenched. The CVD graphene was transferred using conventional wet etching techniques, using a poly(methyl methacrylate) PMMA protective coating and Transene Cu etchant. Graphene films were transferred to SiO 2 (100 nm)/Si substrates, spun dry and baked at 150 °C for 15 min before soaking in acetone for 1 min to remove the PMMA coating. After the transfer process, the graphene sheets were functionalized with either oxygen or fluorine groups using a plasma process, or with hydrogen using the Birch reduction. Oxygen or fluorine moieties were introduced using pulsed electron-beam-generated plasmas. The electron beam is produced by applying a −2-kV pulse to a linear hollow cathode. The beam emerges from the hollow cathode and passes through a slotted anode, and terminates at a second grounded anode located further downstream. The resulting electron beam is magnetically confined, to minimize spreading, producing a sheet-like plasma in background gasses of O 2 /Ar or SF 6 /Ar mixtures to produce the desired functionalities. The system base pressure is maintained at ~1 × 10 −6 Torr before processing by a turbo molecular pump. Reactive gases are introduced at 5% of the total flow rate (180 sccm) with argon providing the balance to achieve an operating pressure of 90 mTorr. For this work, the pulse width was 2 ms and the duty factor was maintained at 10%, O 2 or SF 6 were used as the reactive gas, plasma processing time of 1 min and system pressure of 90 mTorr. All processing was performed at room temperature. Graphene samples were placed on a processing stage adjacent to the plasma at a distance of 2.5 cm from the electron-beam axis. Graphene was hydrogenated via the Birch reduction as described in detail elsewhere [38] . Briefly, substrate-supported graphene was placed in a nitrogen-purged vessel cooled to −78 °C in a dry ice bath. Approximately 10 ml of anhydrous ammonia was distilled into the vessel and 50 mg of lithium metal was added to the liquid in small pieces. Removing the vessel from the cold bath and gently swirling turned the mixture a homogeneous dark blue colour. After 2 min, the reaction was quenched with dropwise addition of 10 ml of ethanol. The graphene was removed from the reaction vessel, rinsed with additional ethanol and dried under nitrogen. Following plasma functionalization, ex-situ XPS measurements using a monochromatic X-ray photoelectron spectrometer (K-Alpha XPS System) with a spot size of 400 μm were performed to assess starting chemical composition (see Supplementary Fig. 9 and Supplementary Methods XPS analysis for more details). All experiments on functionalized graphene sheets were performed within their known lifetimes. Functional groups persist for weeks or months on plasma OG [39] and HG [38] , while the lifetime of FG is on the order of days [40] . To mitigate degradation effects, comparative experiments with fluorinated films were performed within hours of functionalizing the graphene sheets with fluorine. All samples were stored in dry nitrogen when not in use. Experimental setup AFM experiments were performed using an Asylum Research Cypher with an automatic temperature control unit modified to circulate dry nitrogen through the AFM chamber. The ambient temperature was maintained at 29 °C, and O 2 content was measured at <3% within the chamber for all experiments. All experiments were performed with either NSC35 rectangular AFM tips from MikroMasch, with a nominal spring constant of 5.4 N m −1 , AC240TS AFM tips from Olympus with a spring constant of 1 N m −1 , RC800PSA silicon nitride tips from Olympus with a nominal spring constant of 0.76 N m −1 or ultrananocrystalline diamond tips from Advanced Diamond Technologies, Inc. with a spring constant of 0.46 N m −1 . A relationship between cantilever force and vertical deflection was obtained using force–distance curves and thermomechanical noise measurements [41] . These relationships are used to calculate the deflection voltage necessary to apply a specified force. The raw data collected from the experiments were pull-off force, lateral deflection and relative friction as a function of AFM scans and tip load ( Supplementary Fig. 10 ). Bond scission dynamics measurements Friction force was monitored as a function of AFM scan passes within a specified area to measure the chemical dynamics of bond scission during scanning ( Supplementary Fig. 10 ). The AFM tip scans perpendicular relative to the length of the cantilever and measures the relative friction force by taking the difference between the lateral trace and retrace signals. After the first scan, we measure the relative decrease in friction by scanning an area encompassing our original scan area and the unscanned surroundings at low force. The ratio of the friction values between the scanned area and its surroundings provides the calibration between friction signal and relative friction decrease, and is used to calculate the relative friction at all subsequent scans. Another comparison between scanned area and surroundings at the end of the experiment confirms that the ratio is valid throughout the whole experiment. Tip pull-off force measurements after each AFM scan provides one measure of tip wear during the experiment. The adhesion force measured during each force–distance curve is subtracted from the setpoint calculation to prevent underestimating the applied force on the tip. How to cite this article: Felts, J. R. et al . Direct mechanochemical cleavage of functional groups from graphene. Nat. Commun . 6:6467 doi: 10.1038/ncomms7467 (2015).